Direct observation of the three regions in α-synuclein that determine its membrane-bound behaviour α-synuclein (αS) is a protein involved in neurotransmitter release in presynaptic terminals, and whose aberrant aggregation is associated with Parkinson’s disease. In dopaminergic neurons, αS exists in a tightly regulated equilibrium between water-soluble and membrane-associated forms. Here we use a combination of solid-state and solution NMR spectroscopy to characterize the conformations of αS bound to lipid membranes mimicking the composition and physical properties of synaptic vesicles. The study shows three αS regions possessing distinct structural and dynamical properties, including an N-terminal helical segment having a role of membrane anchor, an unstructured C-terminal region that is weakly associated with the membrane and a central region acting as a sensor of the lipid properties and determining the affinity of αS membrane binding. Taken together, our data define the nature of the interactions of αS with biological membranes and provide insights into their roles in the function of this protein and in the molecular processes leading to its aggregation. In the synaptic termini, the 140-residue protein α-synuclein (αS) is partitioned between cytosolic and membrane-associated forms [1] . Although the binding of αS to lipid membranes appears to be implicated in its functional role in synaptic regulation, it may also trigger its aggregation, ultimately leading to the formation of Lewy bodies, which are ubiquitously associated with Parkinson’s disease, one of the most common types of neurodegenerative disorder [2] , [3] , [4] , [5] , [6] , [7] , [8] . Understanding the structure and dynamics of the membrane-bound state of α-synuclein (αS) is therefore a major priority to clarify how for this protein the balance between functional and dysfunctional processes can be regulated. The dynamic nature of αS in both its cytosolic and membrane-bound states has, however, limited the application of standard methods of structural biology, including X-ray crystallography and solution NMR spectroscopy. In its cytosolic form, αS can be monomeric and intrinsically disordered [9] , [10] , [11] or associated with other proteins [12] . Upon binding to lipid membranes, αS undergoes a significant conformational transition with respect to its monomeric intrinsically disordered form, with some regions adopting a high level of α-helical structure [13] , [14] , [15] , [16] . This ordering process is driven by specific amino acid patterns in the αS sequence, in particular those coding for amphipathic class A2 lipid-binding α-helical segments in the region of the molecule spanning residues 1–90 (ref. 16 ). The modular organization of such α-helical fragments promotes αS binding to a wide variety of lipid assemblies, from micelles and lipid vesicles to cellular membranes [14] , [15] , [17] , [18] . As a consequence of its metamorphic character, αS is able to sense membrane curvature and defects, and respond to the presence of specific features such as lipid rafts, adopting a range of structural architectures, such as a pair of antiparallel curved α-helices (residues 3–37 and 45–92) [15] , [17] or a single curved α-helix, encompassing essentially the entire N-terminal region [18] , [19] , [20] . Indeed, NMR studies involving lipids that mimic key features of synaptic vesicles, such as composition and curvature, have revealed that αS binds to lipid bilayers via a multiplicity of distinct binding modes [14] . Taken together, these studies are providing a general view of the structural plasticity and the dynamical nature [21] , [22] , [23] of the membrane-bound state of αS, whose structural properties can sometimes be perturbed even by relatively minor external factors. It is therefore of fundamental importance to study the interactions of αS with lipids under conditions that reproduce as closely as possible the physical properties of presynaptic membranes. Small unilamellar vesicles (SUVs) with appropriate mixtures of DOPE (1,2-dioleoyl- sn -glycero-3-phosphoethanolamine), DOPC (1,2-dioleoyl- sn -glycero-3-phosphocholine) and DOPS (1,2-dioleoyl- sn -glycero-3-phospho- L -serine) lipids have been shown to be excellent models for synaptic vesicles; however, their slow-tumbling rates prevent the detection of most of the signals from bound αS using conventional solution NMR methods [14] . Under these experimental conditions, only resonances from the disordered C terminus, the region of the protein having low membrane affinity, can be detected, while the segment of the protein-containing residues that can interact strongly with membranes is essentially undetectable for solution NMR. In this Communication, we show that it is possible to describe the conformational properties of the elusive membrane-bound state of αS by using a combination of solid-state NMR (ssNMR) spectroscopy and solution NMR chemical exchange saturation transfer (CEST) measurements [24] , [25] , [26] . This approach has proved to be highly effective in enabling the fine tuning between structural order and disorder in the membrane-bound state of αS to be probed directly without requiring any chemical modification of the protein or changes to its amino acid sequence. We find from these studies that αS binds to the membranes of synaptic-like vesicles in such a manner that it generates three different dynamical regimes in distinct regions of the protein sequence. Our combined approach indicates that αS interacts with such vesicles via an α-helical N-terminal ‘anchor’ that also enhances cooperatively the binding of the central region of the sequence to the membrane surface, while the C-terminal region remains largely unstructured and coupled only weakly to the cellular membrane. The central region includes also the ‘non-amyloid-β component’ (NAC) fragment, which has been implicated in the mechanism of αS aggregation, and is here shown to play a key role in modulating the affinity of αS for cellular membranes. We therefore identify an essential region of the amino acid sequence of αS having a role in determining the way the protein partitions between membrane-bound and unbound states as well as in the processes of αS aggregation under pathological conditions leading to Parkinson’s disease. Membrane-bound αS features three distinct regions We used ssNMR to probe the structural properties of αS bound to SUVs that mimic the native composition and curvature of synaptic vesicles [14] . The SUVs utilized in this study are acidic and consist of mixtures of DOPE, DOPS and DOPC in 5:3:2 molar ratios [14] . To characterize the conformational preferences of αS bound to these vesicles, we used a series of magic angle spinning (MAS) ssNMR techniques in conjunction with isotope labelling of the protein, an approach that has been shown to be a powerful means of studying interactions between proteins and membranes [27] , [28] , [29] , [30] , [31] , [32] . A solution of 13 C– 15 N-labelled αS was mixed with DOPE:DOPS:DOPC SUVs, as described previously [14] and in Methods. The resulting vesicles incorporating the labelled αS were subsequently packed into 3.2-mm MAS rotors (Methods). Using circular dichroism (CD), we selected a protein:lipid ratio of 1:65 by monitoring the transition of the protein signal from the disordered state to one with a high degree of α-helical structure, consequent upon addition of lipids ( Supplementary Fig. 1 ). With this protein–lipid ratio, the first 97 residues of αS are effectively invisible with solution NMR techniques because the association of αS with the SUVs broadens dramatically the protein resonances as a result of the slow tumbling of the complex in the absence of a very high degree of internal dynamics, such as that observed in the C-terminal region [14] . To investigate this elusive state, we carried out a series of ssNMR experiments involving 13 C– 13 C dipolar-assisted rotational resonance (DARR) [33] . These spectra correlate both main-chain and side-chain 13 C-labelled resonances of the protein, as a result of cross-polarization (CP) effects, and hence are able to detect rigid moieties of biomacromolecules even in the absence of rapid overall tumbling of the molecule. Indeed, in the study of interactions between proteins and membranes, DARR experiments have been shown to be particularly effective for detecting the resonances of residues that become highly rigid upon interaction with the lipid bilayer, such as, for example, transmembrane α-helices [30] , [34] . Using a DARR contact time of 20 ms, we were able to detect homonuclear correlations between directly bonded carbon atoms in regions of αS that are tightly bound to the membrane ( Fig. 1a,b ). The highest signal intensities in the spectra of the samples studied here were obtained by performing the measurements at −19 °C; that is, under conditions where the lipids adopt a gel phase [35] . Other than having increased signal-to-noise ratios, however, these spectra are fully consistent with those measured at 4 °C. Moreover, no variations in the number of observed resonances or the values of their chemical shifts were observed when the protein:lipid ratios were varied from 1:30 to 1:200. 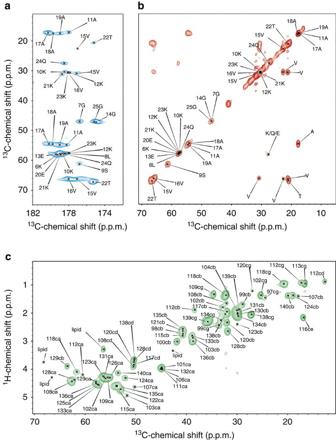Figure 1: MAS ssNMR spectrum of αS bound to DOPE:DOPS:DOPC SUVs. 13C–13C DARR correlation spectrum recorded at −19 °C using a 20 ms contact time at a MAS rate of 10 kHz. Carbonyl and aliphatic regions are shown inaandb, respectively. Residue names are reported using the single letter convention. (c)1H–13C correlation via refocused INEPT transfer recorded at 4 °C at a MAS rate of 10 kHz. The experiments were performed at1H frequencies of 600 and 700 MHz using a1H/13C 3.2-mm probe and a spinning rate of 10 kHz. Atom names ca, cb, cg, cd are used for Cα, Cβ, Cγand Cδatoms, respectively. Figure 1: MAS ssNMR spectrum of αS bound to DOPE:DOPS:DOPC SUVs. 13 C– 13 C DARR correlation spectrum recorded at −19 °C using a 20 ms contact time at a MAS rate of 10 kHz. Carbonyl and aliphatic regions are shown in a and b , respectively. Residue names are reported using the single letter convention. ( c ) 1 H– 13 C correlation via refocused INEPT transfer recorded at 4 °C at a MAS rate of 10 kHz. The experiments were performed at 1 H frequencies of 600 and 700 MHz using a 1 H/ 13 C 3.2-mm probe and a spinning rate of 10 kHz. Atom names ca, cb, cg, cd are used for C α , C β , C γ and C δ atoms, respectively. Full size image DARR experiments performed at a range of different contact times (50, 100, 200 and 500 ms, Supplementary Figs 2 and 3 ) revealed an intense network of dipolar interactions, indicating that the 13 C– 13 C DARR resonances belong to a well-defined structural segment of consecutive residues. The relatively low signal-to-noise ratios did not enable the acquisition of three-dimensional (3D) spectra; however, we were nevertheless able to measure 15 N– 13 C CP correlations ( Supplementary Fig. 4 ) that have provided additional connectivities to those obtained from the 13 C– 13 C DARR spectra. The high redundancy in the αS primary sequence, which includes a series of conserved KTKEGV segments that are repeated imperfectly throughout the N-terminal region, poses a significant challenge for residue-specific assignments. Nonetheless, we were able to assign individual spin systems using 13 C– 13 C DARR spectra recorded at different contact times, in conjunction with heteronuclear correlation experiments ( Supplementary Fig. 4 ) and information from the analysis of the CEST experiments (see below). As a consistency check, the chemical shifts of the assigned resonances were compared with those obtained by solution NMR experiments of αS in SDS and SLAS micelles [17] , [36] . Overall, we have been able to obtain the sequential assignments for the complete segment K 6 GLSKAKEGVVAAAEKTKQG 25 . The ability to observe and assign the resonances of this stretch of the sequence revealed that the N-terminal segment of αS is sufficiently strongly anchored to the membrane to be visible using CP experiments. The measured chemical shift values indicate that this αS segment is in a continuous α-helical conformation when bound to SUVs and, using the δ2D method [37] , we estimate that the population of α-helical structure in this segment is on average 86±11% ( Supplementary Fig. 5 ). In order to probe the effects of lipid composition on the affinity of αS for membranes, we studied the interactions of αS with SUVs consisting of 1-hexadecanoyl-2-(9Z-octadecenoyl)- sn -glycero-3-phospho-(1′-rac-glycerol) (POPG) lipids. αS has been shown to bind strongly to such lipid vesicles [38] and with an affinity that is approximately threefold higher than that found for DOPE:DOPS:DOPC SUVs [19] . This finding is in good agreement with our CD measurements that enabled apparent dissociation constants to be calculated and give values for K d of 93±15 μM for POPG and 261±21 μM for DOPE:DOPS:DOPC SUVs under the conditions employed in the present study ( Supplementary Fig. 1 ). Despite the different binding affinities, however, no significant differences were observed between the DARR spectra of αS bound to POPG ( Fig. 2 ) and those of αS bound to DOPE:DOPS:DOPC vesicles ( Fig. 1a ), indicating that the regions of the protein that are rigid in the membrane-bound state are essentially identical for the two types of SUVs. 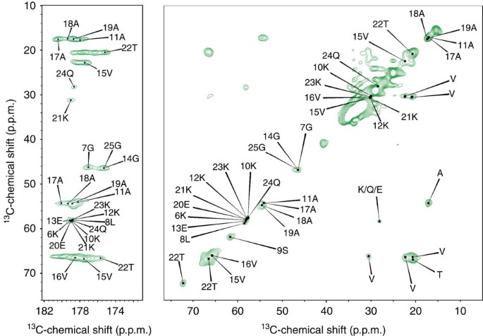Figure 2: MAS ssNMR spectrum of αS bound to POPG SUV. The carbonyl region (left panel) and the aliphatic region (right panel) are shown for the13C–13C DARR correlation spectrum of a sample of αS bound to POPG SUV recorded using a contact time of 100 ms at a temperature of −19 °C and a MAS rate of 10 kHz. Residue names are reported using the single letter convention. Figure 2: MAS ssNMR spectrum of αS bound to POPG SUV. The carbonyl region (left panel) and the aliphatic region (right panel) are shown for the 13 C– 13 C DARR correlation spectrum of a sample of αS bound to POPG SUV recorded using a contact time of 100 ms at a temperature of −19 °C and a MAS rate of 10 kHz. Residue names are reported using the single letter convention. Full size image In addition to the DARR experiments, which provided direct evidence of the regions of αS that are tightly bound to the membranes, insensitive nuclei enhanced by polarization transfer (INEPT) MAS measurements [39] were used to monitor 1 H– 13 C correlations of the most dynamic parts of the protein in the bound state ( Fig. 1c ). Such experiments have been shown to be highly effective probes of regions such as loops in cytoplasmic domains that possess extensive conformational fluctuations relative to those of the more rigid segments of membrane proteins. INEPT spectra of αS bound to DOPE:DOPS:DOPC SUVs showed a significant number of resonances that closely overlap with those observed in solution NMR 1 H– 13 C HSQC spectra of αS in the presence of an excess of SUVs ( Supplementary Fig. 6 ). As the 1 H– 13 C HSQC spectra in solution NMR have been assigned [9] , [14] , comparison of the spectra readily enabled the assignments of the MAS INEPT resonances to be defined ( Fig. 1c ). The resulting assignments correspond to the region 97–140 and indicate that this fragment adopts unstructured conformations in the membrane-bound state. Overall, the MAS measurements indicate three distinct regions in the αS sequence, including a highly rigid N-terminal fragment adopting α-helical conformation, an unstructured C-terminal fragment and a central region, residues 26–96, that adopts an intermediate dynamical regime. Probing the topology of αS bound to lipid bilayers To probe the topology of the membrane-bound state of αS, we employed paramagnetic relaxation enhancement (PREs) experiments [30] . For this purpose, we doped the DOPE:DOPS:DOPC SUVs with low levels (2%) of phosphoethanolamine lipids that incorporate paramagnetic centres in the headgroups or at specific positions in the aliphatic chains [40] . In these experiments, the unpaired electrons from the paramagnetic centres increase the transverse relaxation rates of the nuclei in their vicinity, giving rise to line broadening and hence providing information on the proximity of individual residues of αS to different regions of the lipid bilayers. As a paramagnetic probe, we first used the gadolinium salt of phosphoethanolamine–1,2-dimyristoyl- sn -glycero-3-phosphoethanolamine-N-diethylenetriaminepentaacetic acid (Avanti Polar Lipids Inc.), which carries an unpaired electron on the headgroup. We detected substantial paramagnetic broadening of a subset of resonances in the 13 C– 13 C DARR spectrum of αS bound to SUVs doped with the probe molecule ( Supplementary Fig. 7a ), and observed that hydrophilic residues are significantly more affected than hydrophobic ones. This pattern of behaviour is typical of membrane-associated amphipathic sequences of proteins and peptides that form an α-helix that is bound to the surface of the membrane, such that the hydrophilic residues are located at the water/headgroup interface and the hydrophobic residues are directed towards the inner core of the membrane ( Supplementary Fig. 7c ). Interestingly, we also observed non-negligible attenuations of some of the signals in the 1 H– 13 C INEPT spectrum of αS ( Supplementary Fig. 7b ), including the positively charged K97, the uncharged polar residues Q99 and N103, and the hydrophobic residues L100, A107, I112 and V118. These findings indicate that the C-terminal region of αS interacts weakly and transiently with the membrane surface when bound to SUVs. As these PRE measurements indicate that the N-terminal region of αS lies on the surface of the lipid bilayer, to probe whether or not any part of αS inserts into the interior of the membrane, we used a second paramagnetic agent, 16-doxyl-PC (1-palmitoyl-2-stearoyl-[16-doxyl]- sn -glycero-3-phosphocholine, Avanti Polar Lipids Inc.). This molecule is engineered with a paramagnetic doxyl group at position 16 of the hydrocarbon chain tail, which partitions within the lipid bilayer. We observed no significant paramagnetic relaxation effects on any of the αS resonances bound to SUVs, either in 13 C– 13 C DARR or in 1 H– 13 C INEPT spectra in the presence of this probe ( Supplementary Fig. 8 ). These MAS measurements rule out the possibility that any significant part of αS inserts even transiently into the membrane bilayer. The central region of αS modulates membrane affinity We next carried out a series of CEST experiments [24] , [25] , [26] to gain a deeper understanding of the equilibrium between the unbound and bound states of αS. The CEST approach is an ideal method for probing equilibria between NMR visible (detectable) and invisible (undetectable) states of proteins, including low molecular weight species that are transiently bound to slow-tumbling high-molecular-weight complexes, which indeed cannot be observed directly in solution NMR experiments as a result of excessive line broadening. In the CEST experiments, a continuous weak radiofrequency field is applied off-resonance (by up to 28 kHz) in the 15 N channel, thereby saturating the broad spectroscopic transitions in the bound (undetectable) state but leaving the resonances of the free (detectable) state virtually unperturbed [24] , [25] , [26] . The saturation of the bound state can then be transferred to the free state via chemical exchange, attenuating the intensities of the observable resonances of the latter. By carrying out a series of experiments at various offsets, it is possible to obtain a map of the strength of interactions between the low and high molecular weight species at a residue-specific resolution. In the presence of a small quantity of SUVs (0.06% of lipid mixture, 0.6 mg ml −1 ) all of the αS resonances are detectable in the 1 H– 15 N HSQC spectra, and only marginal changes in the peak intensities are observed. By contrast, substantial differences are observed in CEST experiments ( Fig. 3a and Supplementary Fig. 10 ), which in the presence of SUVs revealed specific resonances from the protein sequence that exhibit strong saturation effects over a broad range of offsets resulting in symmetric CEST profiles ( Fig. 3b ). In probing the interactions between αS and DOPC:DOPE:DOPS SUVs, these experiments show clearly that the strongest saturation effects are observed for residues in the N-terminal region of the protein, indicating that this segment has a tighter association with the SUVs than any other region of the protein ( Fig. 3b ). The saturation effects decrease gradually for residues 26–97 with a sharp transition in the vicinity of residue 98, where the peak intensities of the resonances coincide with those observed in the absence of lipids ( Supplementary Fig. 9 ). These experiments therefore provide a residue-specific measure of the magnitude of the interactions between αS and DOPC:DOPE:DOPS SUVs, and these results are fully consistent with the conclusions of the ssNMR experiments discussed above. Together, these findings reveal that the N-terminal region of αS bound to SUVs forms a stable helix that interacts strongly with the surface of the lipid bilayer, while the C-terminal region of the protein is highly dynamic and motionally independent of the SUVs. 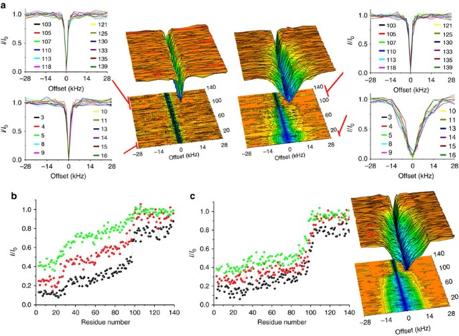Figure 3: CEST experiments probing the membrane-sensor interactions of αS. CEST experiments were recorded at a1H frequency of 700 MHz (see Methods), using a protein concentration of 300 μM and 0.06% (0.6 mg ml−1) of DOPE:DOPS:DOPC lipids in a ratio of 5:3:2 and assembled in SUVs.1H–15N HSQC spectra were recorded by using a continuous wave saturation (170 Hz or 350 Hz) in the15N channel at a range of offsets: −28, −21, −14, −9, −5, −3, −1.5, 0, 1.5, 3, 5, 9, 14, 21 and 28 kHz. An additional spectrum, saturated at −100 kHz, was recorded as a reference. Data recorded using a 350 Hz continuous wave radio frequency are shown (data measured using 170 Hz are reported inSupplementary Fig. 10). (a) CEST surface for the unbound (left) and bound (right) αS; the upper and lower inserts report individual CEST profiles for residues at the N and C termini, respectively. (b) CEST saturation along the αS sequence. Black symbols refer to the averaged CEST profiles measured using offsets at ±1.5 kHz. Similarly, profiles for ±3 and ±5 kHz are shown in red and green, respectively. (c) The interactions between αS and POPG SUVs probed by CEST. Labels as inb. The data were measured using a 350 Hz saturation (seeSupplementary Fig. 11for data acquired using 170 Hz). Figure 3: CEST experiments probing the membrane-sensor interactions of αS. CEST experiments were recorded at a 1 H frequency of 700 MHz (see Methods), using a protein concentration of 300 μM and 0.06% (0.6 mg ml −1 ) of DOPE:DOPS:DOPC lipids in a ratio of 5:3:2 and assembled in SUVs. 1 H– 15 N HSQC spectra were recorded by using a continuous wave saturation (170 Hz or 350 Hz) in the 15 N channel at a range of offsets: −28, −21, −14, −9, −5, −3, −1.5, 0, 1.5, 3, 5, 9, 14, 21 and 28 kHz. An additional spectrum, saturated at −100 kHz, was recorded as a reference. Data recorded using a 350 Hz continuous wave radio frequency are shown (data measured using 170 Hz are reported in Supplementary Fig. 10 ). ( a ) CEST surface for the unbound (left) and bound (right) αS; the upper and lower inserts report individual CEST profiles for residues at the N and C termini, respectively. ( b ) CEST saturation along the αS sequence. Black symbols refer to the averaged CEST profiles measured using offsets at ±1.5 kHz. Similarly, profiles for ±3 and ±5 kHz are shown in red and green, respectively. ( c ) The interactions between αS and POPG SUVs probed by CEST. Labels as in b . The data were measured using a 350 Hz saturation (see Supplementary Fig. 11 for data acquired using 170 Hz). Full size image The CEST experiments were repeated with SUVs prepared with POPG lipids [38] ( Fig. 3c and Supplementary Fig. 11 ). The saturation profiles obtained under these conditions are generally similar to those obtained with DOPC:DOPE:DOPS SUVs, where resonances of residues of the membrane-associated N terminus are strongly affected by off-resonance saturation, while those of the residues of the C terminus are essentially unchanged in intensity. A significant difference in the saturation profiles is, however, found for the central region of the sequence (residues 26–97), which shows much stronger levels of saturation when bound to SUVs composed of POPG lipids ( Fig. 3c ) compared with those observed in the presence of DOPE:DOPC:DOPS SUVs ( Fig. 3a,b ). These data suggest that different regions of αS have distinct roles in the process of association with lipid membranes, such that the N-terminal α-helix (residues 6–25) acts to anchor αS strongly to the membrane, and is only marginally affected by lipid composition, while the region 26–97 appears to act as a membrane ‘sensor’, modulating the strength of the interactions in a lipid-specific manner ( Fig. 4 ). 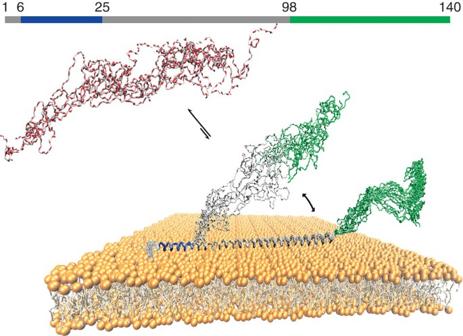Figure 4: Schematic illustration of the different roles of the three regions of αS in determining its interaction with lipid bilayers. We identified three different regimes of protein dynamics and membrane affinity by using a combination of solution and solid-state NMR spectroscopy. The N-terminal region (blue) is visible in DARR experiments, indicating that it is rigidly bound and anchored to the membrane. The central region (grey), showing intermediate dynamics and therefore being invisible in both CP and INEPT experiments, is suggested to play a key role in modulating the affinity of αS for membranes. Finally, a C-terminal fragment (green) maintains its unstructured nature and remains essentially uncorrelated with the membrane surface, despite showing weak and transient contacts in PRE experiments. Figure 4: Schematic illustration of the different roles of the three regions of αS in determining its interaction with lipid bilayers. We identified three different regimes of protein dynamics and membrane affinity by using a combination of solution and solid-state NMR spectroscopy. The N-terminal region (blue) is visible in DARR experiments, indicating that it is rigidly bound and anchored to the membrane. The central region (grey), showing intermediate dynamics and therefore being invisible in both CP and INEPT experiments, is suggested to play a key role in modulating the affinity of αS for membranes. Finally, a C-terminal fragment (green) maintains its unstructured nature and remains essentially uncorrelated with the membrane surface, despite showing weak and transient contacts in PRE experiments. Full size image Although it is now generally recognized that the formation of fibrillar aggregates by αS is a hallmark of Parkinson’s disease, much remains to be understood about the physiological role of this protein [6] . αS possesses an eclectic character and the ability to adopt different conformations resulting in a variety of cytosolic, membrane-bound and aggregated states. In aqueous solutions [9] as well as in cellular milieu [10] , αS has been shown to behave as an intrinsically disordered protein, although there has been evidence for and against the possible existence of more highly structured forms of soluble αS in some environments and in complexes [41] , [42] . Considerable attention has also been focused on the membrane-associated state of αS, which has been suggested to be of great significance in both physiological and pathological contexts. It is indeed evident that αS exists in vivo in an equilibrium between cytosolic and membrane-bound states, with membrane partitioning being tightly regulated [1] , [12] . A particularly intriguing issue in this context is the mechanism by which the affinity of αS to lipid membranes is modulated. There is strong evidence that the population of the bound state is regulated by the intrinsic structural properties of αS and by the composition and the physical properties of the membrane bilayer, such as curvature, charge, packing defects and surface hydrophobicity [15] , [17] , [18] , [36] , [43] . We have explored this fundamental issue by probing the structure and conformational dynamics of αS bound to membranes in its physiological, non-aggregated state. This membrane-bound state is effectively intractable to current X-ray crystallography techniques; however, the success of solution NMR spectroscopy in describing the disordered soluble protein [9] , [10] , [13] , [14] , [15] , [16] , [17] , [36] , [44] , [45] and of solid-state NMR studies in defining the structural properties of the polymorphic forms of the aggregated state of αS [46] , [47] , [48] , [49] prompted us to explore the use of a combination of these techniques to define the structures and dynamics of αS bound in its non-aggregated state to lipid membranes. Our approach can directly probe the interaction with lipid mixtures that mimic those of synaptic vesicles without requiring alterations of the protein sequence or any chemical modification. We have found that, in line with the metamorphic nature of αS [50] , three distinct regions of this protein (the N-terminal, central and C-terminal segments) interact in very different ways with lipid bilayers as a result of their different structural and dynamical properties ( Fig. 4 ). The N-terminal 25 residues, which we denote as the membrane anchor region, adopt a well-defined and highly motionally restricted α-helical conformation that appears to be largely independent of lipid composition. By contrast, the central segment of the protein (residues 26–97), which can be described as a membrane-sensor region, has intermediate dynamical properties. This region is indeed too flexible to be detected by CP experiments but too rigid to be seen by INEPT-type transfer experiments. It is legitimate to assume, however, based on EPR measurements [18] , [20] and transferred NOE data [14] , that this membrane-sensor region adopts α-helical structure when transiently bound to a lipid membrane surface. The present results indicate that the NAC sequence, which has been shown to play a role in the mechanisms of αS aggregation [6] , [51] , [52] , [53] , being included in the membrane-sensor region is also likely to have functional relevance, specifically in defining the affinity of αS for lipid membranes and therefore in modulating the partitioning between membrane-bound and membrane-free states in the synaptic termini. Finally, we have found from PRE experiments that the C-terminal domain (residues 99–140), which has been reported to be highly unstructured and extremely flexible, experiences weak and transient interactions with the membrane surface. In conclusion, by combining solution and solid-state NMR techniques, we have characterized a series of key structural features of the membrane-bound state of αS, and to define the nature of its interactions with lipid assemblies (SUVs) that mimic synaptic-like lipid membranes. From these data has emerged a model to describe the interactions of αS with membranes, which reconciles the results of a range of previous studies [13] , [14] , [15] , [16] , [17] , [18] , [19] , [20] , [36] and also sheds new light on the molecular determinants of binding affinity that are likely to be associated with the physiological role of αS. The nature of these membrane interactions in the processes of αS aggregation underscores the importance of the interplay between different functional states of αS and its aggregation mechanism leading to Parkinson’s disease. αS purification αS was purified in Escherichia coli using plasmid pT7-7 encoding for the protein as previously described [54] . See Supplementary Methods for further details. Preparation of SUVs for solid-state and solution NMR SUVs containing a molar ratio of 5:3:2 of DOPE:DOPS:DOPC (Avanti Polar Lipids Inc.) were prepared from chloroform solutions of the lipids. The lipid mixture was evaporated under a stream of nitrogen gas and then dried thoroughly under vacuum, to yield a thin lipid film. Then the dried thin film was re-hydrated adding an aqueous buffer (20 mM sodium phosphate, pH 6.0) and subjected to vortex mixing. Several freeze-thawing cycles and sonication were carried out until the mixture become clear. In the case of CEST experiments, after sonication, SUVs were mixed with αS samples with a concentration of 0.06% (0.6 mg ml −1 ). In the case of ssNMR experiments, after sonication, αS was added to the SUVs up to a molar ratio of 1:65 protein:lipid. Then the mixture was pelleted at 75,000 r.p.m. for 30 min and 4 °C (Beckman Coulter Optima TLX Inc., USA) by using a rotor TLA 100.3. Subsequently, the SUV-αS sample was transferred to 3.2-mm Zirconia XC thin-walled MAS rotor for the ssNMR experiments. POPG SUV-αS samples were prepared using the same protocol but a solution of 50-mM potassium phosphate buffer and 100-mM NaCl at pH 7.4 was used [19] . MAS measurements All MAS experiments were carried out on either a 14.09T or a 16.85T VNMRS spectrometer with a 3.2-mm BioMASTM probe (Agilent Technologies, USA). DARR experiments [33] were performed at a MAS rate of 10 kHz using different contact times (20, 50, 100, 200 and 500 ms). DARR spectra were acquired at −19 °C and 4 °C (the latter for control experiments only). INEPT experiments were carried out at 4 °C using a MAS rate of 10 kHz. Pulse widths were 2.5 μs for 1 H and 5.5 μs for 13 C, and proton TPPM decoupling was applied at ω RF/(2 π )=71.4–100 kHz. DARR experiments were acquired using a 1-ms CP time and DARR contact times ranging from 50 to 500 ms. Solution NMR samples and CEST experiments Solution NMR experiments were carried out at 10 °C on Bruker spectrometers operating at 1 H frequencies of 700 MHz equipped with triple resonance HCN cryoprobes. CEST experiments were based on 1 H– 15 N HSQC experiments by applying constant wave saturation in the 15 N channel. As the exchange is probed between monomeric αS (having sharp resonances) and the slow-tumbling SUV-bound state (having very broad resonances), a series of large offsets was employed (−28, −21, −14, −9, −5, −3, −1.5, 0, 1.5, 3, 5, 9, 14, 21 and 28 kHz) resulting in CEST profiles of symmetric shape ( Fig. 3a ). An additional spectrum saturated at −100 kHz was recorded as a reference. CEST experiments were performed using two continuous wave radio frequencies (170 and 350 Hz) to saturate 1 H– 15 N-HSQC spectra recorded using a data matrix consisting of 2048 (t 2 , 1 H) × 440 (t 1 , 15 N) complex points. Assignments of the resonances in 1 H– 15 N-HSQC spectra in solution NMR were obtained from previous reports [2] , [9] , [14] . How to cite this article: Fusco, G. et al. Direct observation of the three regions in α-synuclein that determine its membrane-bound behaviour. Nat. Commun. 5:3827 doi: 10.1038/ncomms4827 (2014).